C-C bond cleavage in biosynthesis of 4-alkyl-L-proline precursors of lincomycin and anthramycin cannot precedeC-methylation 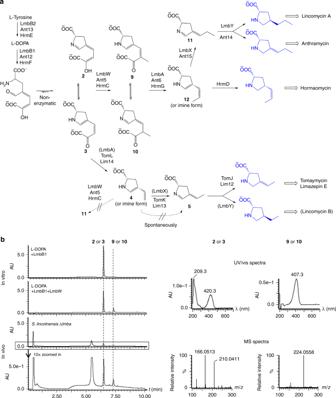Fig. 1 Biosynthetic steps catalyzed by LmbA/Ant6 and LmbW/Ant5 in the context of ALDP pathway.aScheme of ALDP biosynthetic pathway (adopted from Jiraskova et al.2and modified according to Kamenik et al.10); Dotted arrows indicate steps proposed by Zhong et al.1, brackets indicate a side-pathway, final ALDP precursors highlighted in blue are incorporated into the secondary metabolites.bIn vitro (experiments from Jiraskova et al.2re-examined using a more suitable chromatographic method) and in vivo (new experiments)C-methylation of2/3by LmbW; Chromatographic conditions: UPLC BEH Amide 1.7 µm, 2.1 × 50 mm column (Waters, USA), mobile phase: A-acetonitrile and B-50 mM ammonium acetate pH8:acetonitrile 1:1 (v/v), elution: 99% A for 2.5 min followed by a linear decrease from 99 to 1% A in 10 min, UV/VIS chromatograms extracted at 405 nm, MS spectra were recorded using an electrospray ionization technique in a negative mode 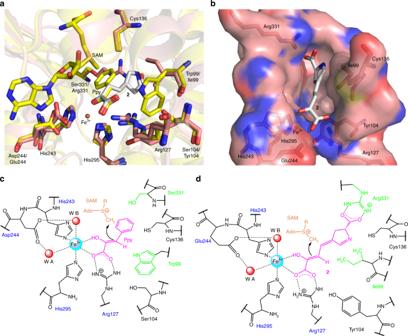Fig. 2 Comparison of the active sites and proposed reaction mechanism of MppJ and LmbW.aComparison of active sites of MppJ (in yellow, crystal structure PDB ID: 4KIC [https://www.rcsb.org/structure/4KIC] with the substrates phenylenolpyruvate (Ppy) andS-adenosyl methionine (SAM)—adopted6) and LmbW (a homology model built using the MppJ structure and the SWISS-MODEL server15); LmbW is in pink; substrate2is in white. The positions of compound2, Fe3+, and SAM in the model were determined by superimposing the model on the 4KIC template in PyMOL16and adjusting the position of2based on the position of the α-keto(enol)-carboxylic moiety of Ppy bound to MppJ.bArrangement of the putative substrate binding pocket with2in the homology model of LmbW.cSchematic active site and a proposed mechanism of action of MppJ6, modified according to panela.dSchematic active site and proposed mechanism of action of LmbW. Panelscandd: abbreviations of residues reflecting the common α-keto(enol)-carboxylic moiety of Ppy and2and the common proposed mechanism are in blue; abbreviations of residues differing in MppJ vs. LmbW, reflecting the uncommon moieties of Ppy vs.2(aromatic ring of Ppy vs. heterocyclic carboxylic moiety of2), are in green. Residue numbering corresponds to MppJ Zhong et al. [1] confirmed that γ-glutamyltranspeptidase (γ-GTs) homologs are capable of cleaving a C–C bond, which was previously inferred by Jiraskova et al. [2] in 2016 in a study based on gene inactivation experiments. The intriguing C–C bond cleavage catalyzed by LmbA and Ant6 γ-GT homologs from the biosynthesis of lincomycin A and anthramycin, respectively, was conclusively documented by Zhong et al. [1] . However, assignment of 2 / 3 as the LmbA and Ant6 substrate and 4 / 5 as the reaction product is questionable for several reasons; most importantly, it contradicts the current state of knowledge of the biosynthesis of 4-alkyl- l -proline derivatives (ALDP or APD used in previous literature; Fig. 1a ) [2] . Here, we argue that LmbA/Ant6 γ-GT homologs do not utilize 2 / 3 , but intermediate 9 / 10 , which was previously proposed to be the main native substrate of LmbA [2] and which is biosynthesized from 2 / 3 by a C -methylation reaction. Consequently, the main LmbA/Ant6 product is not 4 / 5 but compound 12 , which is a subject of isomerization in order to proceed towards the final ALDP of lincomycin A and anthramycin. Fig. 1 Biosynthetic steps catalyzed by LmbA/Ant6 and LmbW/Ant5 in the context of ALDP pathway. a Scheme of ALDP biosynthetic pathway (adopted from Jiraskova et al. [2] and modified according to Kamenik et al. [10] ); Dotted arrows indicate steps proposed by Zhong et al. [1] , brackets indicate a side-pathway, final ALDP precursors highlighted in blue are incorporated into the secondary metabolites. b In vitro (experiments from Jiraskova et al. [2] re-examined using a more suitable chromatographic method) and in vivo (new experiments) C -methylation of 2 / 3 by LmbW; Chromatographic conditions: UPLC BEH Amide 1.7 µm, 2.1 × 50 mm column (Waters, USA), mobile phase: A-acetonitrile and B-50 mM ammonium acetate pH8:acetonitrile 1:1 ( v/v ), elution: 99% A for 2.5 min followed by a linear decrease from 99 to 1% A in 10 min, UV/VIS chromatograms extracted at 405 nm, MS spectra were recorded using an electrospray ionization technique in a negative mode Full size image Here, we bring evidence that 2 / 3 is not the main native substrate of LmbA/Ant6 γ-GT homologs, but of LmbW/Ant5 C -methyltransferases. Indeed, we observed in vitro C -methylation of 2 / 3 by LmbW affording 9 / 10 and we also detected intermediate 9 / 10 in the cultivation broth of the Δ lmbA mutant of lincomycin producing strain Streptomyces lincolnensis (Fig. 1b ). Even though the conversion of 2 / 3 into 9 / 10 by LmbW was only partial, it clearly showed that 2 / 3 serves as an LmbW/Ant5 substrate. To support that conversion of 2 / 3 by LmbW is not a side reaction resulting from broader substrate specificity of LmbW and that its main native substrate is indeed 2 / 3 and not 4 / 5 as the work by Zhong et al. [1] suggests, we carried out a bioinformatic analysis of LmbW/Ant5. We found out that LmbW/Ant5 and their homologs (SibZ [3] , HrmC [4] , and Por10 [5] ) from the biosyntheses of other ALDPs are similar to ALDP-unrelated C -methyltransferases MppJ with known structure [6] and MrsA [7] (26% identity to LmbW according to BLAST for both MppJ and MrsA along the whole sequence; sequence alignment of LmbW and MppJ is available in Supplementary Fig. 1 ). MppJ and MrsA methylate phenylpyruvic and 5-guanidino-2-oxopentanoic acids, respectively, i.e., substrates structurally analogous to 2 / 3 and not 4 / 5 . Furthermore, methylation of phenylpyruvic acid catalyzed by MppJ is part of the biosynthesis of β-methyl- l -phenylalanine from l -phenylalanine [8] . Instead of direct methylation of l -phenylalanine, the machinery requires to proceed via phenylpyruvic acid, indicating the importance of the α-keto(enol)-carboxylic moiety of phenylpyruvic acid for the MppJ-catalyzed methylation. We propose that the same applies also to LmbW/Ant5 because their substrate 2 / 3 also contains the α-keto(enol)-carboxylic moiety. Importantly, conversion of the analogous substrates of MppJ and LmbW/Ant5 through a common reaction mechanism is supported by comparison of the active sites of MppJ (based on the protein crystal structure) [6] vs. LmbW (based on a homology model) depicted in Fig. 2 . The α-keto(enol)-carboxylic moiety appears to play an important role in fixation of the substrate within the active site not only in the case of MppJ, but also LmbW/Ant5. All these enzymes share the residues important for α-keto(enol)-carboxylic moiety fixation as well as the methylation (four residues depicted in blue in Fig. 2c, d ). In contrast to 9 / 10 , intermediate 4 / 5 (proposed as the LmbA/Ant6 reaction product and thus the LmbW/Ant5 substrate by Zhong et al. [1] ) does not possess the α-keto(enol)-carboxylic moiety for the substrate fixation in the active site. Fig. 2 Comparison of the active sites and proposed reaction mechanism of MppJ and LmbW. a Comparison of active sites of MppJ (in yellow, crystal structure PDB ID: 4KIC [ https://www.rcsb.org/structure/4KIC ] with the substrates phenylenolpyruvate (Ppy) and S -adenosyl methionine (SAM)—adopted [6] ) and LmbW (a homology model built using the MppJ structure and the SWISS-MODEL server [15] ); LmbW is in pink; substrate 2 is in white. The positions of compound 2 , Fe 3+ , and SAM in the model were determined by superimposing the model on the 4KIC template in PyMOL [16] and adjusting the position of 2 based on the position of the α-keto(enol)-carboxylic moiety of Ppy bound to MppJ. b Arrangement of the putative substrate binding pocket with 2 in the homology model of LmbW. c Schematic active site and a proposed mechanism of action of MppJ [6] , modified according to panel a . d Schematic active site and proposed mechanism of action of LmbW. Panels c and d : abbreviations of residues reflecting the common α-keto(enol)-carboxylic moiety of Ppy and 2 and the common proposed mechanism are in blue; abbreviations of residues differing in MppJ vs. LmbW, reflecting the uncommon moieties of Ppy vs. 2 (aromatic ring of Ppy vs. heterocyclic carboxylic moiety of 2 ), are in green. Residue numbering corresponds to MppJ Full size image Moreover, the methylation of 4 / 5 would have to proceed through a different mechanism than reactions catalyzed by MppJ and MrsA, which would be inconsistent with the high conservation of the key catalytic residues within the active sites of MppJ and LmbW/Ant5. Based on the above-mentioned arguments, we claim that 2 / 3 is first C -methylated by LmbW/Ant5 and the reaction product 9 / 10 is utilized as a substrate of LmbA/Ant6 γ-GT homologs. However, 2 / 3 can serve as a minor substrate of LmbA if the C -methylation step is omitted and lincomycin B [9] , a side product of lincomycin A biosynthesis, is formed. Similarly, 2 / 3 undergoes C–C bond cleavage if the C- methyltransferase is not encoded within the biosynthetic gene cluster, which applies to the biosynthesis of e.g., tomaymycin [10] , [11] and limazepine E [12] with a two-carbon side-chain ALDP (Fig. 1a ). Therefore, Zhong et al. [1] elucidated the unusual C–C bond cleavage function of LmbA/Ant6, but using other than the main native substrate. Furthermore, Zhong et al. [1] claim that 4 , which they propose to be the product of 2 / 3 cleavage by LmbA/Ant6, is prone to spontaneous isomerization into 5 (Fig. 1a ). They observed this isomerization during their unsuccessful attempt to synthesize 4 . However, 4 was previously synthesized by Saha et al. [13] , it was structurally characterized by nuclear magnetic resonance (NMR) and used for enzymatic assays, but its spontaneous isomerization into 5 was not reported. Specifically, Saha et al. [13] conducted a two-step deprotection of an analogous compound (methyl ester was used instead of tert -butyl ester) using LiOH for methyl ester hydrolysis and trifluoroacetic acid for Boc deprotection, affording 4 , not 5 . Therefore, we consider the formation of 5 during deprotection of 4’ observed by Zhong et al. [1] to be caused by the used deprotecting method. Importantly, spontaneous isomerization of 4 into 5 would be also inconsistent with the function of putative isomerases LmbX/Ant15. They were assigned for enzymatic isomerization of 4 into 5 based on (1) the comparison of the hormaomycin structure and its biosynthetic gene cluster, which does not encode a homolog of LmbX [4] , and (2) the production profile of the Δ lmbX and Δ lmbX Δ lmbW mutants of lincomycin producing strain S. lincolnensis [2] . These data show that if the enzymatic isomerization step of 4 into 5 is not involved in the ALDP biosynthesis, 4 or its analog 12 with a three-carbon side-chain is after reduction of its endocyclic double bond incorporated into the final secondary metabolite. In addition, analytical chemistry data for 5 obtained by Zhong et al. [1] from enzymatic reaction of 2 / 3 with LmbA/Ant6 are not sufficient for unambiguous structural elucidation of this compound. Comparison of 1 H NMR spectra of 5 obtained enzymatically and by chemical synthesis is complicated by partial overlap of the terminal methyl group signal by the signal of NH 4 OAc, which together with a relatively low quality of the spectrum complicates easy identification in the case of the enzymatic product. Without analogous comparison of at least 13 C NMR spectra of 5 obtained from both sources, it is difficult to see their virtual identity. The expansion present in the spectrum of 5 from enzymatic reaction looks like an expansion from a different spectrum. Moreover, the signal at 2.00 ppm (expansion in spectrum a) should be a doublet, similarly as in the spectrum b. Another misleading point is also the chemical name of 5 in page 39 of Supplementary Information , in which its name corresponds to the structure of 4 . In summary, considering also our arguments, work of Zhong et al. [1] represents a crucial missing proof of the ALDP biosynthetic pathway puzzle, i.e., the role of γ-GT homologs in the cleavage of oxalate from 2 / 3 (for compounds with a two-carbon side-chain ALDP) or its methylated derivative 9 / 10 (for compounds with a three-carbon side-chain ALDP including lincomycin A and anthramycin). The subsequent step in anthramycin and lincomycin A biosynthesis presumably involves isomerization catalyzed by LmbX/Ant15 so that the pathway proceeds towards the final ALDP intermediate. [14] Data supporting the findings of this work are available within the paper and its Supplementary Information file and from the corresponding author on request.